Polymorphism of dislocation core structures at the atomic scale Dislocation defects together with their associated strain fields and segregated impurities are of considerable significance in many areas of materials science. However, their atomic-scale structures have remained extremely challenging to resolve, limiting our understanding of these ubiquitous defects. Here, by developing a complex modelling approach in combination with bicrystal experiments and systematic atomic-resolution imaging, we are now able to pinpoint individual dislocation cores at the atomic scale, leading to the discovery that even simple magnesium oxide can exhibit polymorphism of core structures for a given dislocation species. These polymorphic cores are associated with local variations in strain fields, segregation of defects, and electronic states, adding a new dimension to understanding the properties of dislocations in real materials. The findings advance our fundamental understanding of basic behaviours of dislocations and demonstrate that quantitative prediction and characterization of dislocations in real materials is possible. Dislocations, line defects in crystal lattices, and their interactions govern properties of many materials, ranging from fundamental plasticity and work hardening in metals and alloys to device pathology in semiconductor light-emitting and laser diodes or nonvolatile memories [1] , [2] , [3] . In addition, the elastic distortions of regular lattices around dislocations can give rise to a strain field with which the atomic impurities or point defects might interact, forming the so-called ‘Cottrell atmosphere’ that influences many areas of materials science [4] . Technologically, dislocation lines can act as fast pathways for enhanced mass transport, an elemental phenomenon known as pipe diffusion, hence raising an appealing likelihood to synthesize low-dimensional hierarchical nanostructures in crystalline solids for dislocation-engineered devices [5] , [6] . In all these circumstances, whether dislocations are vital or fatal, the atomic-scale structure of their cores, the locus where the lattice planes precisely terminate, assumes paramount importance. Several experimental techniques exist for probing dislocations, but, in general, no one can individually provide sufficient information to constrain a systematic solution to their local core structure at the atomic scale [7] , [8] . X-ray and neutron scattering, as well as electron diffraction, yield a spatially averaged structure and are therefore insensitive to individual defects notwithstanding the increasingly high energy resolution. Although high-resolution atomic force microscopy enables individual dislocations to be identified at the surfaces, it falls short of providing atomic resolution of their cores [9] , impeding a ready inference of their core properties. In contrast, advanced transmission electron microscopy (TEM) is in principle able to directly resolve individual embedded dislocation cores with single-atom sensitivity [10] , [11] , [12] , [13] , particularly in the annular dark-field mode [10] , [11] . This leads to a far greater understanding on the correlation between the dislocation cores in real materials and their mechanical, optical, and electronic behaviours [12] , [14] . Such an understanding is, however, incomplete in that the inherently local TEM imaging can, at best, reveal only a selection of dislocations in real materials, the nature of which is dictated by chemical composition, processing history (for example, mechanical deformation) and geometry of the sample (for example, lattice mismatched thin-film heterostructures) [15] . These substantially complicate our efforts to isolate and hence systematically pinpoint dislocations, thereby posing a relevant yet long unresolved problem in the field of materials science on whether dislocations of an individual type (defined by their characteristic displacement vectors, the Burgers vector b and line vector t ) can take on multiple core structures in real materials at the atomic scale. Addressing this issue has now become likely with the bicrystal technique that allows a precise control over crystallography [16] , [17] , [18] , while diffusion bonding two single crystals to introduce dislocations of a given type. However, the number of possible stable dislocation cores and their corresponding atomic-scale structures are not known in advance. A coherent strategy is therefore indispensable to combine the experimental imaging with comprehensive theoretical simulations in a self-consistent global optimization scheme [19] , [20] . Here we develop such a useful modelling strategy to identify atomic-scale geometries of all dislocation core polymorphs for a prescribed dislocation species (that is, b and t ) in MgO, a prototypical ionic material that finds numerous technological applications where its prevalent dislocations are known or suspected to influence functionality, for example, the tunnel magnetoresistance effect in magnetic tunnel junctions [21] . We demonstrate the power and efficiency of such modelling approach by fabricating MgO bicrystals and directly imaging all predicted dislocation cores with sub-Ångström resolution, providing thereby definitive evidence for the polymorphism of dislocation cores at the atomic scale. By correlating element-selective imaging with the geometrical phase analysis (GPA) and quantum-mechanical calculations, we are able to identify distinct strain fields and local electronic states for the different dislocation cores, which shall have implications for the understanding of many properties and bring a novel dimension to dislocation-engineered materials. Theoretical prediction of dislocation core at the atomic scale Inspired by the bicrystal concept, we build up a periodic array of one-dimensional edge dislocations in MgO by ‘adjoining’ its two single crystals, which are somewhat tilted with respect to each other, while retaining symmetry ( Fig. 1a ). The edge dislocation is chosen because it interacts most strongly with point defects owing to its associated pressure field, which is the key to clarify malfunction mechanisms of many existing devices, while raising hopes for making new ones, for example, straight quantum wires and dots in solids. Such a paradigm for producing dislocations has the advantage of uniquely defining their b and t vectors by manipulating the relative orientations of the two crystals. For example, the crystal orientation in Fig. 1a enables us to harvest dislocations with b = a [100] and t =[110] ( a is lattice constant of MgO). Moreover, the separations between parallel dislocations that are formed at the crystal interface can be precisely adjusted by prescribing the crystal misorientation angle ( θ ) [5] , [17] . 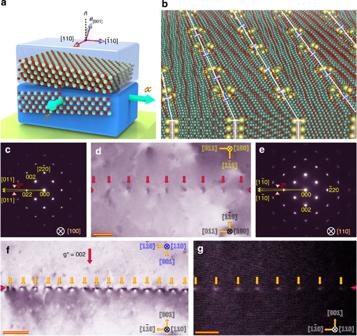Figure 1: Modelling and verification of dislocation array. (a) A one-dimensional edge dislocation array can be generated by adjoining two crystals misoriented about a common axis by a small angleθ. To predict dislocation core structures, we performed an exhaustive search for all core configurations, taking into account the translation of one crystal with respect to the other (depicted by the arrows). The bigger balls in blue represent Mg and the smaller balls in red represent O. (b) Three-dimensionally periodic supercells are constructed for the most stable dislocations and used to perform energy minimization using DFT. The atoms around dislocation cores are highlighted. (c) SADP is taken at the boundary of the (01)[100] bicrystal. (d) A representative cross-sectional bright-field TEM image of the boundary in the (01)[100] bicrystal, viewed along the [100] direction. A periodic image contrast is visible at the boundary area (indicated by arrows), suggesting the existence of embedded dislocation array. Scale bar, 10 nm. (e) SADP taken at the boundary of the (001)[110] bicrystal. (f) A representative bright-field TEM image of the boundary in the (001)[110] bicrystal, viewed from the [110] direction. A periodic image contrast is unambiguously seen as well at the boundary area, inferring the presence of dislocation array. Scale bar, 20 nm. (g) Low-magnification ADF STEM image of the boundary in the (001)[110] bicrystal, confirming the presence of a periodic one-dimensional dislocation array at the boundary. Scale bar, 10 nm. Figure 1: Modelling and verification of dislocation array. ( a ) A one-dimensional edge dislocation array can be generated by adjoining two crystals misoriented about a common axis by a small angle θ . To predict dislocation core structures, we performed an exhaustive search for all core configurations, taking into account the translation of one crystal with respect to the other (depicted by the arrows). The bigger balls in blue represent Mg and the smaller balls in red represent O. ( b ) Three-dimensionally periodic supercells are constructed for the most stable dislocations and used to perform energy minimization using DFT. The atoms around dislocation cores are highlighted. ( c ) SADP is taken at the boundary of the (01)[100] bicrystal. ( d ) A representative cross-sectional bright-field TEM image of the boundary in the (01)[100] bicrystal, viewed along the [100] direction. A periodic image contrast is visible at the boundary area (indicated by arrows), suggesting the existence of embedded dislocation array. Scale bar, 10 nm. ( e ) SADP taken at the boundary of the (001)[110] bicrystal. ( f ) A representative bright-field TEM image of the boundary in the (001)[110] bicrystal, viewed from the [110] direction. A periodic image contrast is unambiguously seen as well at the boundary area, inferring the presence of dislocation array. Scale bar, 20 nm. ( g ) Low-magnification ADF STEM image of the boundary in the (001)[110] bicrystal, confirming the presence of a periodic one-dimensional dislocation array at the boundary. Scale bar, 10 nm. Full size image To predict atomic-scale structure of dislocations in the bicrystal, we construct atomistic models of symmetric low-angle boundaries between two 10 nm-thick MgO crystals in the direction normal to interface ( Fig. 1a ), and impose periodic boundary conditions parallel to interface. Interactions between ions are described by classical polarizable interatomic potentials [22] that are very accurate and efficient for ionic materials, thereby allowing an exhaustive search for stable interfaces by minimizing total energies with respect to ion coordinates and translation of one grain relative to the other ( Fig. 1a ). Such a procedure in general yields a series of metastable boundary structures involving different dislocation cores, their relative stability of which can be accessed by comparing interface formation energy defined as E f =( E (bicrystal)— N MgO E coh )/ A , where E (bicrystal) is the energy of the bicrystal; E coh is the cohesive energy of bulk MgO; N MgO is the number of MgO units; and A is the interface area [23] . For a range of uncovered low-formation energy bicrystals, we create three-dimensionally periodic supercells containing dislocation dipoles and perform a structural energy minimization using density functional theory (DFT) calculations ( Fig. 1b ). In virtue of finite barriers to dislocation motion, we are able to acquire stable dislocation structures, despite that mutual interaction between dislocations may lead to their eventual annihilation. Validation of bicrystal modelling approach To address specific cases, we consider first the b = a /2[110] edge dislocation in the slip system of MgO, which is the most stable and has been investigated previously, thereby offering a useful validation to our approach. 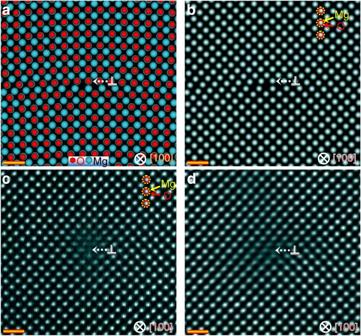Figure 2: Sole type of dislocation core in the slip system. (a) Predicted model of an edge dislocation withb=a/2[110], viewed from [100] direction. The arrows indicate the core location. Note that a systematic modelling uncovers only one dislocation core species in the primary slip system. (b) Simulated HAADF STEM image using the predicted core model. The dotted circle in yellow indicates Mg column and the dotted one in red indicates O column. The Mg and O columns are overlapped from [100] direction. (c,d) Atomic-resolution HAADF STEM (c) and HRTEM (d) images taken from [100] direction, which match the predicted model and associated simulated images well. It is noteworthy that many regions in several TEM samples have been explored and only one dislocation core type has been found. Scale bar, 5 Å. Figure 2a shows a predicted structure of the a /2[110] dislocation core, which represents the only stable one by a systematic search. A mirror plane is preserved passing through the dislocation core area, and this core holds an inconsiderable excess volume, as also revealed in simulated high-angle annular dark-field (HAADF) scanning TEM (STEM) image using the predicted model ( Fig. 2b ). Importantly, this dislocation core contains a string of fivefold under-coordinated ions at the tip of extra half-plane of atoms, in contrast to the sixfold coordination in the bulk MgO, resulting in a deformation of the octahedra close to the core and hence local property shift [24] . Figure 2: Sole type of dislocation core in the slip system. ( a ) Predicted model of an edge dislocation with b = a /2[110], viewed from [100] direction. The arrows indicate the core location. Note that a systematic modelling uncovers only one dislocation core species in the primary slip system. ( b ) Simulated HAADF STEM image using the predicted core model. The dotted circle in yellow indicates Mg column and the dotted one in red indicates O column. The Mg and O columns are overlapped from [100] direction. ( c , d ) Atomic-resolution HAADF STEM ( c ) and HRTEM ( d ) images taken from [100] direction, which match the predicted model and associated simulated images well. It is noteworthy that many regions in several TEM samples have been explored and only one dislocation core type has been found. Scale bar, 5 Å. Full size image To test this predicted core structure, we fabricate a bicrystal with the bicrystallographic relations (01)[100] upper || (01)[100] lower ( Supplementary Fig. 1 ), that is, two crystals are sliced exactly along (01) plane of MgO lattice and the two finely polished surfaces are solid-state diffusion bonded with [100] direction of the upper crystal almost parallel to [100] direction of the lower one by a small tilt angle of θ =1°. Analysis of selected area diffraction pattern (SADP) taken at the boundary confirms these orientations to within the prescribed misfit tilt angle of ~0.84° estimated upon the splitting spots in the pattern ( Fig. 1c ), and the TEM characterization reveals a perfect joining with dislocations periodically aligned along the boundary (indicated by arrows in Fig. 1d ). Further comprehensive g *· b analysis ( g * is the diffracting reciprocal lattice vector) of the dark-field images taken at a series of imaging conditions pinpoints that these dislocations are of edge type with b = a /2[110] ( Supplementary Fig. 2a,c ). Upon closer inspection using Cs-corrected HAADF and annular bright-field (ABF) [25] STEM, as well as high-resolution TEM (HRTEM), we obtain a direct structural imaging of dislocation cores at atomic resolution, albeit the fact that their accompanying strain fields may remarkably blur lattice images. The bright spots in the HAADF STEM image represent the normal MgO atomic columns ( Fig. 2c ), unravelling a core geometry that is in line with the simulated HAADF STEM image using the predicted atomic model ( Fig. 2b ). Such a configuration is further verified in the ABF STEM ( Supplementary Fig. 3b,c ) and HRTEM images ( Fig. 2d ) in which the comprehensive image simulation recognizes the bright spots as sites of atomic columns ( Supplementary Fig. 4a ). We also conduct an atom-resolved imaging of the dislocations at many other boundary regions in several TEM specimens, and find interestingly that all acquired images point to identical core geometry, thereby providing a solid validation of our method. Polymorphism of dislocation core structures In addition to the a /2[110] dislocation, we extend the developed modelling strategy to systematically search core geometries of the b = a [100] edge dislocation, which has been discovered in MgO subjected to high-temperature electricfield treatment [26] . This dislocation has long been deemed as a culprit for catastrophic failure of the intrinsically insulating properties of MgO, yet a clear understanding of its thermal-electric breakdown still poses crucial challenges owing to the lack of atomistic detail of its cores. Based upon an exhaustive theoretical search by taking into account full ion optimization, translations of one crystal with respect to the other and addition and removal of ions at interface, as well as by calculating their associated formation energies, we predict three species of a [100] dislocation core configurations ( Fig. 3a–c ) with similar formation energies (1.7–2.4 J m −2 ), in contrast to the sole type found for the a /2[110] dislocation (0.89 J m −2 ). The dislocation core that is predicted to be most stable, that is, having lowest E f of 1.71 J m −2 (named type I), consists of a fairly open and symmetric core [27] , and remains stable with respect to the insertion of additional atoms in the void ( Fig. 3a ), for example, adding four extra atomic columns raises E f to 1.97 J m −2 . The somewhat less stable dislocation core with a E f of 2.13 J m −2 (named type II) contains a pair of climb partial dislocations (that is, bearing less than a unit lattice translation vector) bounding a stacking fault of ~1.5 nm (cores are indicated by the arrows in Fig. 3b ). In fact, we find interestingly a series of stable type II dislocations, which display varying spacings between the two partials, while imposing little impact on their formation energies. In contrast to the type I dislocation, the dislocation core with highest E f of 2.39 J m −2 (named type III) turns more compact and hence induces heavier strain in the surrounding lattice ( Fig. 3c ). Structurally, it is considered as resulting from the two partial dislocations close together until ultimately a spatial symmetry is formed. 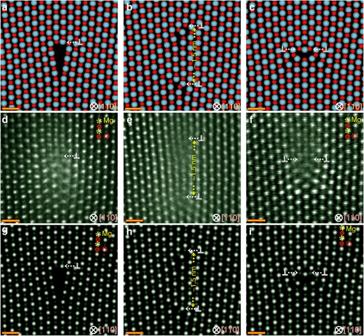Figure 3: Polymorphism of dislocation cores at the atomic scale. (a–c), Three models are predicted for thea[100] dislocations: a singleb=a[100] dislocation with no splitting (type I) (a); twob=a/2[100] partial dislocations bounding a stacking fault of ~1.5 nm (type II) (b); and a singleb=a[100] dislocation with splitting (type III) (c). The three core structures differ locally from one another, albeit the fact that they share the same Burgers vector, thereby underscoring the importance in identifying each individual core structures for even a single dislocation. (d–f) HAADF STEM images of the type I (d), II (e), and III (f) dislocations taken from [110] direction, consistent with the predicted atomic models both geometrically and in quantity. The Mg columns (indicated by larger circles) are distinguishable from O columns (indicated by smaller circles) along the [110] direction. Special care has been taken with the imaging because the strain fields associated with the cores may blur the images. (g–i) Simulated HAADF STEM images of thea[100] dislocations obtained using the predicted models: type I (g), II (h) and III (i) dislocations. Scale bar, 5 Å. Figure 3: Polymorphism of dislocation cores at the atomic scale. ( a – c ), Three models are predicted for the a [100] dislocations: a single b = a [100] dislocation with no splitting (type I) ( a ); two b = a /2[100] partial dislocations bounding a stacking fault of ~1.5 nm (type II) ( b ); and a single b = a [100] dislocation with splitting (type III) ( c ). The three core structures differ locally from one another, albeit the fact that they share the same Burgers vector, thereby underscoring the importance in identifying each individual core structures for even a single dislocation. ( d – f ) HAADF STEM images of the type I ( d ), II ( e ), and III ( f ) dislocations taken from [110] direction, consistent with the predicted atomic models both geometrically and in quantity. The Mg columns (indicated by larger circles) are distinguishable from O columns (indicated by smaller circles) along the [110] direction. Special care has been taken with the imaging because the strain fields associated with the cores may blur the images. ( g – i ) Simulated HAADF STEM images of the a [100] dislocations obtained using the predicted models: type I ( g ), II ( h ) and III ( i ) dislocations. Scale bar, 5 Å. Full size image To verify the prediction that the a[100] dislocations show polymorphism at the atomic scale, we again rely on the geometry-tunable bicrystal technique to prepare boundaries with bicrystallographic relations (001)[110] upper || (001)[110] lower ( Supplementary Fig. 1 ). The pre-designated orientations with a small misfit tilt angle of θ =~1° are testified in the diffraction pattern ( Fig. 1e ), ensuring a successful introduction of an array of dislocations aligned periodically at boundary, as seen in the TEM and STEM images ( Fig. 1f,g ). Upon a comprehensive g *· b analysis, these dislocations are pinpointed as edge ones with an identical Burgers vector b = a [100] ( Supplementary Fig. 2 ). Further atomic-resolution imaging of individual dislocation at many boundary areas leads to a surprising conclusion that all of the probed dislocations eventually fall into three categories as revealed in the HAADF STEM images ( Fig. 3d–f ). The brighter spots in the HAADF images represent Mg columns, whereas lighter ones represent O columns, outlining the three core configurations that match elegantly with their predicted atomic models and simulated HAADF images ( Fig. 3g–i ). To add further support, we also acquire the atomic-resolution ABF STEM and HRTEM ( Supplementary Figs 3 and 5 ) images for the three predicted dislocation cores, in good accord with their simulated counterparts using the three predicted models ( Supplementary Fig. 4b–d ), thereby providing unequivocal evidence that various core polymorphs do exist for even a single-dislocation species at the atomic scale. The power and efficiency of such a complex modelling strategy can be further demonstrated by a direct atom-resolved imaging of a complementary type II dislocation core involving the two partials separated further apart ( Supplementary Fig. 6 ), in strong support of the theoretical predictions. For over five decades, TEM has enabled individual dislocations to be imaged, resulting in a much improved understanding of the interplay between defect structures of materials and their properties. Some of the traditional views, however, may need to be reconsidered, as the resulting implications rest more on a selective imaging than on a comprehensive atomic characterization. Such calling for a reinterpretation of existing structure–property relationships should now become particularly imminent because the current discovery of core polymorphism at the atomic scale adds instantly a novel dimension to the established characterization scheme that highlights the effect of dislocations with different b and t vector [28] . It should be noted that for very low-angle grain boundaries where dislocations are separated well enough to be considered isolated, that is, dislocation cores are surrounded by regions of perfect crystal, such dislocation core polymorphism cannot be simply represented by structural multiplicity of grain boundaries ( Supplementary Discussion ). This first (to our knowledge) finding in MgO also takes on practical significance in nanoelectronic devices where miniaturization immediately requires a priori knowledge of dislocation core structures in that they are often associated with notably different strain fields, tendencies to accumulate defects or impurities and local electronic states, all of which dominate device functionalities. To quantify local differences and shed light on the consequence of core polymorphism, we first perform a GPA of the aberration-corrected HRTEM images to assess strain fields associated with the dislocations [29] , a quantity responsible for many phenomena in material science. The aberration corrector is harnessed to suppress substantially lattice distortions in a conventional HRTEM image arising from projection lens, thereby allowing a precise displacement measurement at the atomic level. The strain field ( ε xx ) is spatially localized (~3 nm) and relies heavily on specific dislocation cores ( Fig. 4a–d ), underscoring the relevance in unravelling all cores for one dislocation type at the atomic scale. It is noteworthy that our calculated dislocation interval (~12 nm) is much longer than the characteristic radius of the associated dislocation strain field (~3 nm) indicating that the dislocations are separated to such a degree that they can be viewed isolated. Dislocations in our very low-angle grain boundaries can hence be considered to represent bulk lattice dislocations and have an equivalent core structure ( Supplementary Discussion ). Interestingly, the a /2[110] and type III a [100] dislocations can give rise to a typical compression-tension strain field pair at their cores, whereas the others display an extra converse butterfly-tie-like pair region in between, which may provide varying driving force for impurity segregation towards dislocations. This scenario can be verified in the summed electron energy-loss spectra acquired from both the bulk and core area showing segregation of Ca and Ti to the three otherwise impurity-free a [100] dislocations, yet no impurity segregation at all to the a /2[110] dislocation ( Supplementary Fig. 7 ). The presence of Ca at the cores is not surprising, given that it is the majority impurity in MgO (ref. 30 ), is isovalent, and exhibits a strong segregation tendency owing to the ion-size misfit effect. The Ti impurity, however, may be either introduced unintentionally during the surface treatments of the MgO single crystals and fabrication of the bicrystals or segregated from the MgO bulk, although it is not detectable in the bulk. Such presence of Ti could be because of the space charge of the dislocation cores or as a result of either thermodynamics (that is, enhanced segregation) or kinetics (that is, enhanced diffusion) effect. The different ability to trap impurities or defects may account for the thermal-electric breakdown in MgO sample where a large amount of a [100] dislocations are formed [26] . 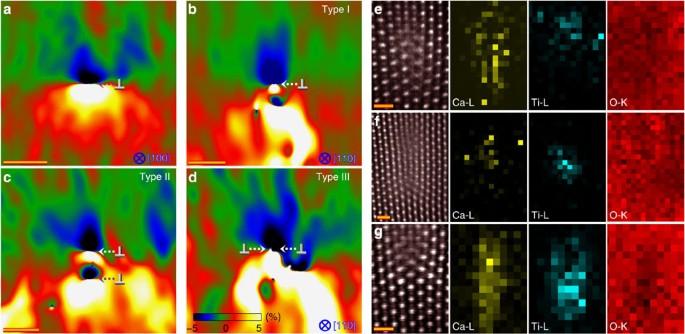Figure 4: Local property shift for polymorphic dislocation cores. (a–d) Strain maps of the in-planeεxxcalculated by the GPA for thea/2[110] (a) and the type I (b), II (c) and III (d)a[100] dislocations. The GPA is performed using the obtained aberration-corrected HRTEM image. Thexandydirections are predefined as [01] and [011] for thea/2[110] dislocation, whereas as [001] and [10] for thea[100] dislocations, respectively. The colour bar indicates change in strain intensity from –5.0% (compressive) to 5.0% (tensile). Scale bar, 2 nm. (e–g) Magnified HAADF STEM images and core-loss images of the Ca-L2,3, Ti-L2,3and O-K edges viewed from [110] direction for the type I (e), II (f) and III (g)a[100] dislocations. Core-loss images are made where the HAADF STEM images are taken. Scale bar, 5 Å. Figure 4: Local property shift for polymorphic dislocation cores. ( a – d ) Strain maps of the in-plane ε xx calculated by the GPA for the a /2[110] ( a ) and the type I ( b ), II ( c ) and III ( d ) a [100] dislocations. The GPA is performed using the obtained aberration-corrected HRTEM image. The x and y directions are predefined as [01] and [011] for the a /2[110] dislocation, whereas as [001] and [10] for the a [100] dislocations, respectively. The colour bar indicates change in strain intensity from –5.0% (compressive) to 5.0% (tensile). Scale bar, 2 nm. ( e – g ) Magnified HAADF STEM images and core-loss images of the Ca-L 2,3 , Ti-L 2,3 and O-K edges viewed from [110] direction for the type I ( e ), II ( f ) and III ( g ) a [100] dislocations. Core-loss images are made where the HAADF STEM images are taken. Scale bar, 5 Å. Full size image Figure 4e–g shows two-dimensional electron energy-loss spectra maps of the Ca-L 2,3 , Ti-L 2,3 and O-K edges by focusing on the core area of a [100] dislocations. Ca prefers to segregate to the dilated part of edge dislocation in that it is oversized in Mg substitution, while size-comparable Ti resides at either compressive or tensile region depending on the specific core type and segregation circumstance [30] . Oxygen is, however, uniformly distributed regardless of the dislocation core type. Apart from the different spatial segregation behaviour, the multiple cores are accompanied by characteristic discrepancies in electronic properties as well, as our DFT calculations reveal qualitatively new gap states for all the four dislocation cores even in the absence of impurities, which vary with dislocation core types ( Supplementary Fig. 8 ). These gap states clearly originate from the defective structures at the dislocation core, that is, both under-coordination of ions and local strain. Further analysis of interatomic bond length at the core reveals that it varies substantially at the core area, and the degree of variation depends heavily on specific core species as well ( Supplementary Fig. 9a–d ). However, the interatomic bonding at the core maintains ionic nature as in the case of bulk MgO, irrespective of the different core species, as shown in the isosurface plots of charge density ( Supplementary Fig. 9e–h ). The close match of predicted dislocation cores with direct imaging both geometrically and in quantity offers confidence that the modelling approach represents a reliable routine to pinpointing all core configurations for even a given dislocation type at the atomic scale. Such ability should afford new perspectives on dislocation activities that have hitherto been explored either selectively or in average, providing therefore a basis for inferring the dislocation-related mechanisms and for designing the dislocation-engineered devices. The finding that dislocation cores can exhibit multiple structures and local property variations promises to advance our understanding on properties of MgO including the abnormal rise in electrical conductivity. Such a modelling paradigm that allows atomic-scale resolving of dislocation core polymorphism is general and should be applicable to many complex materials in which the behaviour of dislocation cores is decisive to understand a range of properties. Calculational process and methodology The dislocation core structures were predicted using the theoretical bicrystal approach implemented in the METADISE code [31] . It involved constructing a two-dimensionally periodic interface between two grains that were oriented at any prescribed angles ( Supplementary Fig. 1a ). The grains were modelled with periodic boundary conditions parallel to interface and were sufficiently wide along interface normal, such that relevant properties and interface formation energies were converged. In the calculations presented here, each crystal was as thick as 10 nm in the direction normal to interface. Interactions between ions in the bicrystal were described by polarizable interatomic potentials [22] that have been shown to be accurate and efficient for many ionic materials. Ions within 4 nm of the interface were allowed to relax, whereas more distant ions were held fixed at their bulk sites. It is noteworthy that this approach is in principle not limited to such potentials. Recent advances in the charge equilibration potentials [32] , [33] and linear-scaling DFT [34] could open the way to applying this modelling approach to more complex crystals including impurity segregation. Structures of the bicrystals were fully optimized with respect to the positions of ions near the interface, rigid translation of one crystal with respect to the other, and addition and removal of ions at the interface. Such a procedure in general yielded a series of boundary structures involving different dislocation cores, the relative stability of which could be assessed by comparing interface formation energy defined as E f =( E (bicrystal)— N MgO E coh )/ A , where E (bicrystal) was the energy of bicrystal; E coh was the cohesive energy of bulk MgO; N MgO was the number of MgO units; and A was the interface area. For the most stable inequivalent bicrystal structures, we had created three-dimensionally periodic supercells containing two dislocation dipoles, which were fully optimized using the GULP code. DFT calculation The supercells served as initial models for further DFT calculations using Vienna ab initio simulation package [35] . We applied the projector augmented-wave method [36] with 4 × 1 × 1 k- point grids and a cutoff energy of 400 eV, which enabled an accurate prediction of both atomic and electronic structures of the dislocation systems. Dislocation cores were modelled with large periodic supercells containing up to 1,600 atoms using the DFT, which were adopted further for the image simulations. All atoms in the supercells were fully optimized until the magnitude of force on every atom converged to <0.05 eV per Å, yielding optimized structures. It is worth mentioning that DFT calculations retain the dislocation core structures predicted by the classical polarizable interatomic potentials, thereby validating the application of these potentials to predict dislocation cores in ionic oxide MgO. In addition, it should be noted that electronic structures of every dislocation core have been calculated using the DFT in order to reveal the electronic difference between the discovered dislocation cores. Bicrystal sample fabrication Two classes of MgO bicrystals with a small tilt angle of θ =1° were prepared by the bicrystal technique by joining two pristine single-crystal blocks (upper and lower) of MgO (purity: 99.9%, Shinkosha, Tokyo): one had the bicrystallographic relationships of (01)[100] upper || (01)[100] lower and the other (001)[110] upper || (001)[110] lower , as sketched in Supplementary Fig. 1a . The size of each single-crystal block was set to be 10 × 10 × 5 mm 3 and thus 10-mm cubic bicrystals were produced. To fabricate the predesigned bicrystals with the confined dislocation arrays, the two single crystals were first cut precisely along (01) (or (001)) plane of MgO lattices, followed by mechanical grinding and polishing of the two contacting planes to mirror finish with diamond slurry of 0.25 μm. Next, the two revealed surfaces were bonded face to face with the [100] (or [110]) direction of one crystal almost parallel to the [100] (or [110]) direction of the other by the small tilt angle of ~1° under hot pressing at 1,773 K for 10 h in air. The picture of final bicrystal was given in Supplementary Fig. 1b , in which dislocations were expected to lie at the boundary region indicated by arrows. The heating and cooling rates were set to be 300 K h −1 during pressing. Several slices with a dimension of 10 × 10 × 1.5 mm 3 were cut from the final bicrystal blocks to prepare specimens for TEM and STEM observations. TEM specimen preparation and imaging condition Thin-foil TEM and STEM specimens were prepared by first cutting slices from the final bicrystal blocks along (011) (or (10)) plane. The slices were then mechanically ground till their thickness reached ~0.12 mm, which was followed by a further dimpling down to ~20 μm. To make electron transparent, the dimpled slices were finally thinned by argon-ion sputter beam using PIPS 691 (Gatan Co., Ltd.). A gun voltage of 1–4 kV and an incident beam angle of 4–6° were used in order to avoid, to maximum extent, radiation damage to the sample. SADPs, TEM and HRTEM images were taken using the JEOL JEM-2010F and FEI TITAN80-300 electron microscopes equipped with image corrector. The HAADF and ABF images were taken with the 200-kV JEM-2100F and ARM-200FC STEM, both of which were equipped with a probe corrector (CEOS Gmbh), providing thereby unprecedented opportunity to probe structures with sub-Ångström resolution. For the HAADF STEM imaging, a probe convergence angle of ~22 mrad and a detector with an inner semi-angle of over 60 mrad were adopted. ABF STEM images were made with a 6–25 mrad detector, and electron energy-loss spectra was recorded using a Gatan Enfina system equipped on the STEM with an energy resolution, at full-width of half-maximum, of ~0.5 eV. Image simulation and GPA Both HRTEM and HAADF STEM image simulations were performed using the commercially available WinHREM package (HREM Research Inc.), which was based upon the multislice method. The fully optimized atomic models obtained from the DFT calculations were adopted for image simulations. The spherical and chromatic aberration coefficients were assumed as C s =0.7 mm and C c =1.6 mm, respectively, to simulate the HRTEM images. The 200-kV probe was assumed to have a probe-forming aperture of 22 mrad and the ADF annular detector was adopted to span the range of 81–228 mrad. Debye–Waller factor was taken into account for each element involved, yet was averaged over spatial directions, namely, the anisotropy of the absorption of thermal diffuse scattering factors was ignored in the image simulations. The GPA [29] , [37] was performed based on the aberration-corrected HRTEM images using a GPA plug-in package (HREM Research Inc.), which was implemented in the Digital Micrograph software (Gatan). How to cite this article: Wang, Z. et al. Polymorphism of dislocation core structures at the atomic scale. Nat. Commun. 5:3239 doi: 10.1038/ncomms4239 (2014).